APC/C is an essential regulator of centrosome clustering Centrosome amplification has been extensively associated with cancer. Cancer cells with extra centrosomes have the ability to cluster the extra centrosomes and divide in a bipolar fashion. Although a number of proteins have been shown to be involved in centrosome clustering, a mechanistic understanding of how this process is coordinated is not yet well defined. Here, to reveal regulators of centrosome clustering, we perform small interfering RNA (siRNA) screens with multiple assay readouts in a human isogenic cellular model. We find that APC/C activity is essential for centrosome clustering. We show that the motor kinesin Eg5 is a substrate of APC/C-CDH1, and that inhibition of APC/C results in stabilization of Eg5. Increased Eg5 protein levels disturb the balance of forces on the spindle and prevent centrosome clustering. This process is completely reversed after a short treatment with the Eg5 inhibitor, monastrol. These data advance our understanding of the regulation of centrosome clustering. Centrosomes serve as microtubule organizing centres in animal cells and have a key role in organizing the mitotic spindle. Efficient bipolar spindle assembly requires coordination of centrosome and DNA replication. Therefore, centrosome duplication is precisely controlled during the cell cycle where it takes place only once during S-phase in a semi-conservative fashion [1] . Cancer cells often fail to tightly control centrosome numbers, which results in supernumerary centrosomes, a feature that has long been associated with cancer. In order to form a bipolar spindle, cancer cells are likely to cluster extra centrosomes in a bipolar fashion during mitosis, thereby preventing deleterious multipolar divisions, in a process termed centrosome clustering [2] . Although this mechanism is associated with defects, such as missegregation, that lead to chromosomal instability, it is essential for the survival of cells with centrosome amplification (CA) [3] , [4] . A number of studies in mammalian and Drosophila models have described proteins and protein complexes that are associated with centrosome clustering, many of them being involved in the organization of microtubules [5] , actin cytoskeleton and cell adhesion [4] and the chromosomal passenger complex [6] . The anaphase-promoting complex/cyclosome (APC/C) is an essential E3 ligase involved in regulating mitotic progression. APC/C activation and substrate selectivity are carefully controlled at different stages of the cell cycle via its co-activator subunits CDC20 and CDH1, which recruit substrates to the APC/C and are essential for its enzymatic activity [7] , [8] . CDK1 is one of the major regulators of co-activator binding to APC/C. In particular, during early mitosis, CDC20 is phosphorylated by CDK1, thereby allowing APC/C-CDC20 to be activated once the spindle assembly checkpoint (SAC) has been satisfied. At the same time, CDK1 phosphorylation of CDH1 prevents association of the APC/C with CDH1. Until anaphase onset, the SAC prevents activation of the APC/C-CDC20 complex. When the SAC is satisfied, APC/C-CDC20 is allowed to target its substrates, such as cyclin B and Securin for degradation, and thereby allows anaphase onset. Once cyclin B is degraded, CDK1 is inactivated and CDH1 is allowed to associate with the APC/C and direct its activity until late G1 phase of the cell cycle [8] , [9] . Here we show for the first time that APC/C-CDH1 is an essential regulator of centrosome clustering. To elucidate the mechanisms underlying centrosome clustering and to identify potential novel targets for therapy in CA cancer cells, we used a synthetic approach, that is, a spindle morphology phenotypic assay by high-content microscopy and a cell viability assay followed by functional protein association analysis. We used a custom-made siRNA ‘spindle- and centrosome-associated’ library and the human siRNA ‘kinome’ library to find siRNAs that induce multipolar spindles specifically in CA cells but not tetraploid or diploid cells with normal centrosome number. This approach, among other hits, allowed the identification of robust target genes that cause cell lethality specifically through multipolar mitosis and only in cells with CA. The knockdown of several APC/C subunits showed a robust multipolar phenotype in our screens, specifically in CA cells. We show that induction of spindle multipolarity as a result of APC/C inhibition is dependent on activity of motor kinesin Eg5, and that Eg5 protein stability is regulated by APC/C-CDH1. In addition, we describe a model where increased Eg5 protein levels impair the ability of the cells to cluster supernumerary centrosomes. Generation and characterization of the cellular model The cellular model that we adopted is based on the generation of chromosomally stable human colon adenocarcinoma DLD1 diploid (2N) and tetraploid (4N) cells, along with tetraploid CA (4NCA) cells ( Fig. 1a and Supplementary Fig. 1a,b ). In order to generate 4NCA cells, we used dihydrocytochalasin B (DCB) to transiently block cytokinesis and induce tetraploidization and CA in DLD1 cells. Shortly after the release (4 h) from DCB, >95% of 4NCA cells had increased centrosome numbers; the majority (>70%) of cells clustered the extra centrosomes during mitosis forming a bipolar spindle, often in an asymmetrical manner ( Supplementary Fig. 1e ). These cells retained high percentage of CA for at least 7 days after the release from DCB. However, they did not retain CA after prolonged culturing, suggesting the existence of mechanisms that reduce the extra centrosomes (possibly by asymmetrical clustering) while the DNA content remains stable ( Supplementary Fig. 1f ). To generate stable 2N and 4N cells, DLD1 were treated with DCB and allowed to grow for several days into stable cell populations before sorting them according to cell cycle profile into diploid (2N) and tetraploid (4N) populations. Comparative genomic hybridization did not show differences between 2N and 4N cells. In addition, 4N cells did not become aneuploid even after prolonged culturing ( Supplementary Fig. 1a,b ) and did not show significant differences in gene expression ( Supplementary Fig. 1c,d ). Growth rate examination of the generated isogenic cell lines showed a slower proliferation of the 4NCA population compared with 2N and 4N cells, possibly because of a longer activation of the SAC in order to allow time for microtubule attachment and centrosome clustering ( Supplementary Fig. 1c ). To validate the quality performance of our cellular model, we used siRNA toward the kinesin KIFC1 and the compound griseofulvin (GSF) as controls. Both approaches showed centrosome de-clustering and increased toxicity against 4NCA cells ( Supplementary Fig. 2a–c ). 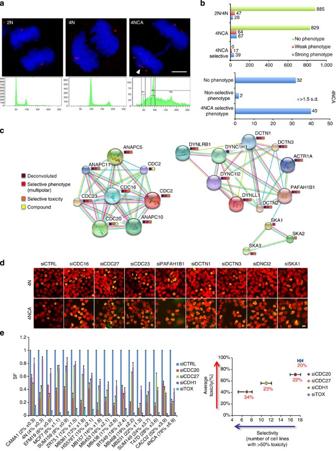Figure 1: siRNA screening and validation. (a) Cell cycle profile of diploid (2N), tetraploid (4N) and tetraploid with centrosome amplification (4NCA) cells. Representative immunocytochemistry images of anaphase cells stained with centriolar marker CP110 (red) and DNA using DAPI (blue). Scale bar, 5 μm. Arrow indicates centriole clustering. (b) Graphical representation of the number of siRNAs that induced multipolar phenotypes in 2N/4N and 4NCA cells (top), and the siRNAs that induced selective toxicity in 4NCA cells categorized by the presence of multipolar phenotype (bottom). (c) Hit and near hit protein clusters generated by STRING database. Coloured boxes indicate hit validation by siRNA pool deconvolution and/or chemical compounds where available. (d) Immunocytochemistry images of 4N and 4NCA cells transfected with siRNAs toward the indicated hit genes. Cells were stained using Aurora A antibody (green) and propidium iodide (red). Scale bar, 5 μm. (e) Left panel, surviving fraction (SF) assays in a panel of 18 cell lines following knockdown of the indicated genes. In parentheses, the percentage of CA. Error bars and±indicate s.d. from at least three different experiments. Right panel, average toxicity of the indicated siRNAs across the cell line panel is plotted (yaxis) against the number of cell lines (xaxis) that showed more than 50% toxicity by the respective siRNA. Red numbers represent average percentage of CA; horizontal bars indicate range. Figure 1: siRNA screening and validation. ( a ) Cell cycle profile of diploid (2N), tetraploid (4N) and tetraploid with centrosome amplification (4NCA) cells. Representative immunocytochemistry images of anaphase cells stained with centriolar marker CP110 (red) and DNA using DAPI (blue). Scale bar, 5 μm. Arrow indicates centriole clustering. ( b ) Graphical representation of the number of siRNAs that induced multipolar phenotypes in 2N/4N and 4NCA cells (top), and the siRNAs that induced selective toxicity in 4NCA cells categorized by the presence of multipolar phenotype (bottom). ( c ) Hit and near hit protein clusters generated by STRING database. Coloured boxes indicate hit validation by siRNA pool deconvolution and/or chemical compounds where available. ( d ) Immunocytochemistry images of 4N and 4NCA cells transfected with siRNAs toward the indicated hit genes. Cells were stained using Aurora A antibody (green) and propidium iodide (red). Scale bar, 5 μm. ( e ) Left panel, surviving fraction (SF) assays in a panel of 18 cell lines following knockdown of the indicated genes. In parentheses, the percentage of CA. Error bars and±indicate s.d. from at least three different experiments. Right panel, average toxicity of the indicated siRNAs across the cell line panel is plotted ( y axis) against the number of cell lines ( x axis) that showed more than 50% toxicity by the respective siRNA. Red numbers represent average percentage of CA; horizontal bars indicate range. Full size image siRNA screening and hit validation In order to find siRNAs that kill CA cells by inducing multipolar spindles, we used two readout assays, a viability assay and a spindle morphology (phenotypic) assay. Based on phenotypic assays, 67 genes in total when ablated, induced a strong multipolar phenotype in 4NCA cells ( Fig. 1b top graph); of these, 28 genes induced strong phenotype also in 2N/4N cells, possibly due to cytokinesis failure or centrosome over-duplication. Based on viability assays, 74 genes in total showed selective toxicity in 4NCA cells ( Fig. 1b bottom graph); 40 of these genes also showed multipolar phenotype selectively in 4NCA cells. The most significant genes that are selective toward CA 4NCA cells, which were confirmed in separate assays by deconvolution of the original siRNA pools, are shown in Tables 1 and 2 . In parallel, to reveal closely associated hits we performed connectivity analysis and K-means clustering of the primary hits, using STRING [10] at default settings. Next, we combined the connectivity map generated by STRING with the siRNA deconvolution data. Genes that were closely clustered and induced multipolar phenotype in 4NCA cells but not in 2N or 4N cells (named ‘Selective phenotype’), as well as selective toxicity against 4NCA cells (named ‘Selective toxicity’), were favoured for further investigation ( Fig. 1c and Supplementary Fig. 2d ). Based on this approach, three major clusters of genes were revealed such as the E3 ubiquitin ligase APC/C subunits, the dynein/dynactin complex (as previously shown [5] ) and the SKA1, 2, 3 complex ( Fig. 1c,d and Supplementary Fig. 2d–f ). Table 1 Results of parallel siRNA screen (phenotypic/viability) of the human kinome library. 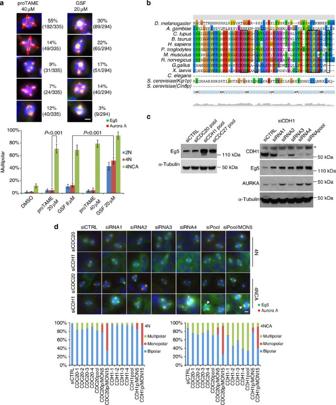Figure 2: Inhibition of APC/C induces distinct multipolar phenotype that is associated with increased Eg5 protein levels. (a) Representative immunocytochemistry images of 4NCA cells (top) and percentage of multipolar phenotypes (bottom) of 2N, 4N and 4NCA cells after treatment with the indicated concentrations of proTAME or GSF; cells were stained for Aurora A (red), Eg5 (green) and DNA using DAPI (blue). Arrows illustrate rotational symmetry. Scale bar, 5 μm. In parentheses, the number of mitotic cells with the indicated phenotype versus the total number of mitotic cells measured.P-value derived from unpaired two-tailedt-test. Error bars represent s.d. from five different experiments. (b) Alignments of full-length Eg5 protein sequences; frames show conserved KEN and D-box APC/C recognition motifs across different species. (c) Immunoblot assays in lysates from 2N cells transfected with the indicated pools or individual siRNAs. Asterisk indicates non-specific band. (d) Immunocytochemistry images of 4N and 4NCA cells transfected with the indicated siRNAs (pool and individual). siRNA pool-transfected cells were additionally treated with the indicated concentrations of monastrol. Cells were stained using specific antibodies against Eg5 (green), Aurora A (red) and DAPI for DNA (top). Scale bar, 5 μm. Quantification of bipolar, multipolar and monopolar spindles (n=>150 mitoses/condition; bottom). Arrows indicate mitotic cells treated with siRNA pools±monastrol. Full size table Table 2 Results of parallel siRNA screen (phenotypic/viability) of the spindle- and centrosome-associated custom library. Full size table We extended our hit validation using siRNAs toward the APC/C subunit CDC27 and the two known co-activators CDC20 and CDH1 in a panel of cancer cell lines encompassing models with varying levels of CA ( Fig. 1e and Supplementary Fig. 3a ). We categorized the siRNAs according to the following two criteria: (a) average reduction of surviving fraction across the panel (toxicity) and (b) number of cell lines with >50% reduction of surviving fraction (selectivity). Knockdown of CDH1 showed the highest selectivity (7/18 cell lines) in contrast to CDC20 that was the least selective of the three (17/18 cell lines). Importantly, the group of cell lines sensitive to CDH1 knockdown contained the highest average CA (34%; Fig. 1e ). However, siCDH1 did show a degree of toxicity overall that can be attributed either to other functions of CDH1 or to the genetic background of the cell lines. Although these data indicate that APC/C regulates centrosome clustering and the formation of bipolar spindle in CA cells, the actual ‘effector’ protein, which is regulated by APC/C, remained unknown. We observed that the spindle morphology induced by APC/C knockdown or treatment with the APC/C-CDC20/CDH1 inhibitor proTAME [11] , [12] showed a well-structured threefold or fourfold rotational symmetry and the spindle poles clearly located at the periphery of the DNA ( Figs 1d and 2a ; and Supplementary Fig. 3a ). In contrast, in multipolar phenotypes induced by small molecule compounds or siRNAs that interfere with microtubule function (for example, GSF [13] ) or cytokinesis (for example, ESPL1), this symmetry is uncommon ( Fig. 2a and Supplementary Fig. 3b ). Furthermore, at higher concentrations, GSF induced multipolar spindles even in cells without CA ( Fig. 2a ). In contrast, proTAME did not induce any multipolar phenotype at any concentration in cells without CA ( Fig. 2a ). This suggests that APC/C inhibition acts in a specific manner to induce multipolar spindles in CA cells. Figure 2: Inhibition of APC/C induces distinct multipolar phenotype that is associated with increased Eg5 protein levels. ( a ) Representative immunocytochemistry images of 4NCA cells (top) and percentage of multipolar phenotypes (bottom) of 2N, 4N and 4NCA cells after treatment with the indicated concentrations of proTAME or GSF; cells were stained for Aurora A (red), Eg5 (green) and DNA using DAPI (blue). Arrows illustrate rotational symmetry. Scale bar, 5 μm. In parentheses, the number of mitotic cells with the indicated phenotype versus the total number of mitotic cells measured. P -value derived from unpaired two-tailed t -test. Error bars represent s.d. from five different experiments. ( b ) Alignments of full-length Eg5 protein sequences; frames show conserved KEN and D-box APC/C recognition motifs across different species. ( c ) Immunoblot assays in lysates from 2N cells transfected with the indicated pools or individual siRNAs. Asterisk indicates non-specific band. ( d ) Immunocytochemistry images of 4N and 4NCA cells transfected with the indicated siRNAs (pool and individual). siRNA pool-transfected cells were additionally treated with the indicated concentrations of monastrol. Cells were stained using specific antibodies against Eg5 (green), Aurora A (red) and DAPI for DNA (top). Scale bar, 5 μm. Quantification of bipolar, multipolar and monopolar spindles ( n =>150 mitoses/condition; bottom). Arrows indicate mitotic cells treated with siRNA pools±monastrol. Full size image Monastrol reverses multipolarity induced by APC/C inhibition We hypothesized that Eg5 represents a strong candidate substrate of APC/C based on two reasons. First, Eg5 cross-links and slides microtubules [14] , thereby generating outward forces that are antagonized by dynein-dependent inward forces [15] . Depletion of dynein/dynactin subunits in our assays generated multipolar spindles in 4NCA cells ( Fig. 1d ), whereas as expected [16] , [17] , Eg5 depletion or inhibition induced primarily monopolar spindles ( Fig. 2d ). In addition, cells where Eg5 is overactive often undergo multipolar mitosis [18] . Second, Eg5 carries several putative KEN [19] and D-box [20] motifs at the C-terminal. In particular, the KEN and D-box motifs at 1,022–1,024 and 1,047–1,050 (RLPL) amino acids, respectively, are in close proximity to promote cooperative binding [21] and, importantly, these motifs are highly conserved among different species ( Fig. 2b ). Based on the above observations, we performed a series of experiments to investigate whether Eg5 is regulated by the APC/C and whether this regulation is essential for centrosome clustering. Knockdown of CDH1 and CDC27 resulted in increased Eg5 protein levels ( Fig. 2c ). Furthermore, knockdown of CDH1 selectively induced multipolar spindles in 4NCA cells but not in 2N ( Supplementary Fig. 4a ) or 4N cells ( Fig. 2d ). This effect was completely reversed by low concentrations of monastrol (5 μM; Fig. 2d ). CDC20 knockdown showed a weak effect on multipolar spindle formation and Eg5 expression ( Fig. 2d graph; and Supplementary Fig. 4b ). These data indicate that primarily CDH1 depletion induces multipolar phenotype in an Eg5-dependent manner. To further investigate the contribution of APC/C-CDH1 and APC/C-CDC20 in centrosome clustering, we inhibited APC/C at different phases of the cell cycle. In asynchronous cells, proTAME, unlike GSF (20 μM) and taxol (0.5 μM), specifically induced multipolar spindles in 4NCA cells. This effect was reversible by short monastrol treatment at low concentrations ( Fig. 3a and Supplementary Fig. 5a ). Similar experiments were performed in cells immediately after release from nocodazole. proTAME treatment caused only a modest increase of multipolar spindles, in contrast to GSF that induced the same strong multipolar phenotype in both, nocodazole treated or asynchronous cells ( Fig. 3b and Supplementary Fig. 5a ). Interestingly, inhibition of APC/C or protein degradation by MG132, solely in mitosis, did not reproduce the phenotype observed in asynchronous cells by proTAME. Also, treatment with proTAME from S-phase until mitosis did not fully reproduce the multipolar spindle phenotype observed in asynchronous cells ( Supplementary Fig. 5b ). Finally, to investigate the effect of APC/C inhibition from anaphase onset for a complete cell cycle, we treated 4N and 4NCA cells with proTAME or GSF after release from a sequential thymidine, nocodazole and MG132 arrest. Following treatment, >80% of 4NCA cells treated with proTAME showed centrosome de-clustering that was reversible by monastrol ( Fig. 3c and Supplementary Fig. 5a,c ). All data together indicate that APC/C-CDH1 inhibition is the major contributor to multipolar spindle phenotype in comparison with APC/C-CDC20, most likely by regulating Eg5 protein stability. 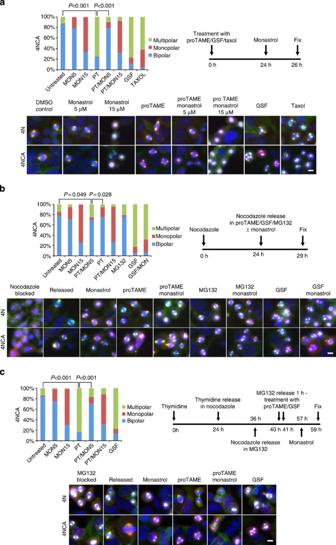Figure 3: Effect of APC/C inhibition at different phases of the cell cycle in spindle multipolarity. (a) Immunocytochemistry images of asynchronous 4N and 4NCA cells after treatment with the indicated compounds. (b) Cells were released from nocodazole block in the presence of the indicated compounds. (c) 4N and 4NCA cells were treated with the indicated compounds after sequential arrest in thymidine, nocodazole and MG132. Scale bar, 5 μm. Quantification of bipolar, multipolar and monopolar mitoses in 4NCA cells (graphs;n=>120 mitoses/condition/experiment,P-value derived from unpaired two-tailedt-test; (a,b) five different experiments; (c) three different experiments). GSF, griseofulvin (20 μM), PT, proTAME; MON, monastrol. Schematics of the treatment regimen used to assess the effect of the indicated compound treatment on spindle phenotype in 4N and 4NCA cells are shown for each experiment. Figure 3: Effect of APC/C inhibition at different phases of the cell cycle in spindle multipolarity. ( a ) Immunocytochemistry images of asynchronous 4N and 4NCA cells after treatment with the indicated compounds. ( b ) Cells were released from nocodazole block in the presence of the indicated compounds. ( c ) 4N and 4NCA cells were treated with the indicated compounds after sequential arrest in thymidine, nocodazole and MG132. Scale bar, 5 μm. Quantification of bipolar, multipolar and monopolar mitoses in 4NCA cells (graphs; n =>120 mitoses/condition/experiment, P -value derived from unpaired two-tailed t -test; ( a , b ) five different experiments; ( c ) three different experiments). GSF, griseofulvin (20 μM), PT, proTAME; MON, monastrol. Schematics of the treatment regimen used to assess the effect of the indicated compound treatment on spindle phenotype in 4N and 4NCA cells are shown for each experiment. Full size image Protein stability of Eg5 is regulated by APC/C In co-localization experiments, Eg5 localization, as expected, followed that of Aurora A, a known APC/C-CDH1 substrate [22] that persisted on the spindle and mitotic bridge in proTAME-treated cells ( Fig. 4a ). Examination of the total protein levels of Eg5 in different phases of the cell cycle revealed that Eg5 is low in G1 and peaks in mitosis, similarly to Aurora A ( Fig. 4b top left). Furthermore, proTAME treatment stabilized Eg5 and Aurora A protein levels in G1 in cells forced to exit mitosis by CDK1 inhibition (CGP74514) and induced accumulation of both proteins in G2 ( Fig. 4b top right). In order to examine whether the putative KEN and D-box motifs ( Fig. 2b ) influence stability of Eg5 protein in cells, we transfected cells with green fluorescent protein (GFP) tagged wild-type Eg5 (WTEg5-GFP) or a truncated form of Eg5 (1-951aa; ΔCEg5-GFP) in which the KEN and D-box motifs at the C terminus of the protein are deleted and GFP-positive cells were isolated by fluorescence-activated cell sorting (FACS) for downstream analysis ( Supplementary Fig. 6 ). Notably, the truncated C-terminal fragment of ΔGCEg5-GFP contains the conserved KEN and D-box motifs and one putative D-box motif that is not conserved. Examination of Eg5-GFP protein levels in mitotic cells and immediately after mitosis showed that WTEg5-GFP is regulated in a similar manner to endogenous Eg5 protein. In contrast, in ΔCEg5-GFP or WTEg5-GFP cells treated with proTAME, exogenous Eg5 remains stable after exit from mitosis ( Fig. 4b bottom, and Supplementary Fig. 7a ). To confirm these results, we introduced point mutations in the KEN and D-box motifs in WTEg5-GFP (DKEg5-GFP) construct. All three Eg5 constructs (WTEg5-GFP, ΔCEg5-GFP and DKEg5-GFP) localized at the mitotic spindle as expected ( Fig. 4c top). In addition, after transient DCB treatment of ΔCEg5-GFP cells, DKEg5-GFP cells and cells that express WTEg5-GFP at much higher levels than those of endogenous Eg5 (WTEg5-GFP high) showed reduced viability and higher frequency of multipolar mitoses relative to cells that express low levels of WTEg5-GFP ( Fig. 4c bottom). Importantly, WTEg5-GFP co-immunoprecipitated with endogenous CDH1 and CDC27 in cells that have been released from mitotic block ( Fig. 5a and Supplementary Fig. 7c ). In contrast, ΔCEg5-GFP co-immunoprecipitated with endogenous CDH1 and CDC27 significantly less. The weak pulldown of CDH1 and CDC27 by ΔCEg5-GFP may be attributed to the association of the truncated protein to endogenous Eg5. Importantly, WTEg5-GFP is ubiquitinated in MG132 treated cells that are forced to exit mitosis by inhibiting CDK1, whereas this ubiquitination is lost in the presence of proTAME ( Fig. 5b top). Moreover, purified Eg5-FLAG (bottom) is ubiquitinated in vitro by APC/C-CDH1 ( Fig. 5b bottom and Supplementary Fig. 7b ). These data together indicate that Eg5 is a true substrate of APC/C-CDH1. It is known that APC/C targets motor kinesins for degradation. KIF18A in mammalian cells and Cin8 and Kip1 in yeast have been shown to be targeted for ubiquitination and degradation by APC/C-CDH1 (refs 23 , 24 , 25 , 26 ). Notably, Kip1 is the closest yeast homologue of Eg5, and Cin8 is considered the yeast orthologue of Eg5. However, pairwise protein alignment of Kip1 or Cin8 shows weight matrix score (ClustalW2) of 26.6 and 23.4, respectively. In addition, homology of the yeast motors to the human Eg5 is mostly in the kinesin motor domains, which are highly conserved across many species. In contrast, the C-terminal regions of vertebrate Eg5 proteins, where we have identified the functional KEN and D-box motifs ( Fig. 2b ), do not show significant sequence homology to the yeast motor kinesins. Therefore, we show for the first time that Eg5 protein is directly regulated by APC/C. 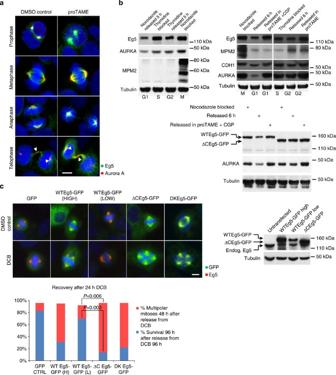Figure 4: Expression of Eg5 lacking C-terminal KEN and D-box motifs or overexpression of wild-type Eg5 induces spindle multipolarity. (a) Representative images of untreated parental DLD1 cells (2N) or treated with 30 μM proTAME, in prophase, metaphase, anaphase and telophase as detected by immunocytochemistry using specific antibodies against Eg5 (green) and Aurora A (red). DNA was stained with DAPI (blue). Scale bar, 5 μm. Arrows indicate co-localization of Eg5 with Aurora A. (b) Eg5 protein levels across the cell cycle in DLD1 cells (2N) were detected by immunoblotting using a specific Eg5 antibody (top left). Eg5, CDH1 and Aurora A protein levels across the cell cycle in the presence of proTAME or proTAME with CGP74514 were detected by immunoblotting using the indicated antibodies (top right). Eg5 and Aurora A protein levels in WTEg5-GFP or truncated ΔCEg5-GFP-expressing cells that were released from nocodazole block in growth media alone or in the presence of proTAME with CGP74514 were detected by immunoblotting using the indicated antibodies. Aurora A is used as CDH1 substrate control, MPM2 as mitotic marker and α-tubulin as loading control (bottom). (c) DMSO-treated control DLD1 cells (2N) and DCB-released DLD1 cells (4NCA) expressing high or low levels of WTEg5-GFP, truncated ΔCEg5-GFP or D-KEN point mutant DKEg5-GFP were analysed for Eg5 localization by immunocytochemistry using specific antibodies toward GFP and Eg5. Scale bar, 5 μm (top left). Stacked column chart showing the percentage of survival (blue) and multipolar mitosis (red) in DCB-released cells expressing high or low levels of WTEg5-GFP, ΔCEg5-GFP or DKEg5-GFP. Survival is shown at 96 h after release from DCB treatment relative to untreated GFP control cells (blue). Multipolar mitoses are shown at 48 h after release of all samples from DCB (red;n≥200 mitoses/condition/experiment,P-value derived from unpaired two-tailedt-test, five different experiments; CTRL, control cells; bottom). Immunoblot shows exogenous Eg5 protein levels relative to endogenous (Endog.) Eg5 as indicated (top right). Figure 4: Expression of Eg5 lacking C-terminal KEN and D-box motifs or overexpression of wild-type Eg5 induces spindle multipolarity. ( a ) Representative images of untreated parental DLD1 cells (2N) or treated with 30 μM proTAME, in prophase, metaphase, anaphase and telophase as detected by immunocytochemistry using specific antibodies against Eg5 (green) and Aurora A (red). DNA was stained with DAPI (blue). Scale bar, 5 μm. Arrows indicate co-localization of Eg5 with Aurora A. ( b ) Eg5 protein levels across the cell cycle in DLD1 cells (2N) were detected by immunoblotting using a specific Eg5 antibody (top left). Eg5, CDH1 and Aurora A protein levels across the cell cycle in the presence of proTAME or proTAME with CGP74514 were detected by immunoblotting using the indicated antibodies (top right). Eg5 and Aurora A protein levels in WTEg5-GFP or truncated ΔCEg5-GFP-expressing cells that were released from nocodazole block in growth media alone or in the presence of proTAME with CGP74514 were detected by immunoblotting using the indicated antibodies. Aurora A is used as CDH1 substrate control, MPM2 as mitotic marker and α-tubulin as loading control (bottom). ( c ) DMSO-treated control DLD1 cells (2N) and DCB-released DLD1 cells (4NCA) expressing high or low levels of WTEg5-GFP, truncated ΔCEg5-GFP or D-KEN point mutant DKEg5-GFP were analysed for Eg5 localization by immunocytochemistry using specific antibodies toward GFP and Eg5. Scale bar, 5 μm (top left). Stacked column chart showing the percentage of survival (blue) and multipolar mitosis (red) in DCB-released cells expressing high or low levels of WTEg5-GFP, ΔCEg5-GFP or DKEg5-GFP. Survival is shown at 96 h after release from DCB treatment relative to untreated GFP control cells (blue). Multipolar mitoses are shown at 48 h after release of all samples from DCB (red; n ≥200 mitoses/condition/experiment, P -value derived from unpaired two-tailed t -test, five different experiments; CTRL, control cells; bottom). Immunoblot shows exogenous Eg5 protein levels relative to endogenous (Endog.) Eg5 as indicated (top right). 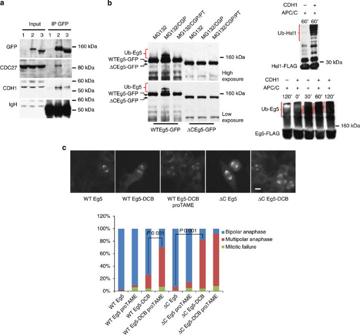Figure 5: Eg5 pulls down CDH1 and CDC27 and is ubiquitinated by APC/C-CDH1. (a) WTEg5-GFP and ΔCEg5-GFP were immunoprecipitated from cells using a rabbit α-GFP antibody. α-GFP, α-CDC27 or α-CDH1 antibodies were used for immunoblotting. α-CDH1 membrane was re-probed with a goat α-rabbit antibody; (1) empty vector (GFP), (2) WTEg5-GFP, and (3) ΔCEg5-GFP. (b) Immunoblot of WTEg5-GFP, ΔCEg5-GFP cells released from nocodazole block in MG132, MG132/CGP74514 or MG132/CGP74514/proTAME (left);in vitroubiquitination assay using purified human APC/C with purified human CDH1 and purified human Eg5-FLAG or yeast Hsl1 as substrates (right). The length of incubation under each condition is indicated in minutes. (c) Still frames of cells treated with the indicated compounds (top; scale bar, 5 μm) and quantification of bipolar anaphases (blue), multipolar anaphases (red) and mitotic failure (green) in cells expressing WTEg5-GFP or truncated ΔCEg5-GFP (graph; bottom;n≥150 concluded mitoses/condition/experiment,P-value derived from unpaired two-tailedt-test, four different experiments). Full size image Figure 5: Eg5 pulls down CDH1 and CDC27 and is ubiquitinated by APC/C-CDH1. ( a ) WTEg5-GFP and ΔCEg5-GFP were immunoprecipitated from cells using a rabbit α-GFP antibody. α-GFP, α-CDC27 or α-CDH1 antibodies were used for immunoblotting. α-CDH1 membrane was re-probed with a goat α-rabbit antibody; (1) empty vector (GFP), (2) WTEg5-GFP, and (3) ΔCEg5-GFP. ( b ) Immunoblot of WTEg5-GFP, ΔCEg5-GFP cells released from nocodazole block in MG132, MG132/CGP74514 or MG132/CGP74514/proTAME (left); in vitro ubiquitination assay using purified human APC/C with purified human CDH1 and purified human Eg5-FLAG or yeast Hsl1 as substrates (right). The length of incubation under each condition is indicated in minutes. ( c ) Still frames of cells treated with the indicated compounds (top; scale bar, 5 μm) and quantification of bipolar anaphases (blue), multipolar anaphases (red) and mitotic failure (green) in cells expressing WTEg5-GFP or truncated ΔCEg5-GFP (graph; bottom; n ≥150 concluded mitoses/condition/experiment, P -value derived from unpaired two-tailed t -test, four different experiments). Full size image Eg5 overexpression induces multipolar spindles in CA cells Next we performed time-lapse experiments to examine the kinetics of centrosome clustering and to verify that the phenotype observed in proTAME-treated or ΔCEg5-expressing cells following DCB release is not an over-represented transient state in fixed cells. We found that <25% of DCB-released cells that express low levels of WTEg5-GFP cells underwent multipolar anaphase, whereas proTAME-treatment increased the fraction of the same cells undergoing multipolar anaphase to >60%. In contrast, in ΔCEg5-GFP cells under the same conditions >70% of the cells went through multipolar anaphases. proTAME treatment or expression of ΔCEg5-GFP in DCB-released cells resulted in prevention of clustering and consequently led to an increase in multipolar anaphases ( Fig. 5c and Supplementary Movies 1–5 ). Under both conditions, multiple centrosomes were unable to migrate in a bipolar fashion during prophase or cluster in metaphase, thus confirming the pivotal role of Eg5 in this process. A model for spindle multipolarity In metaphase of cells with CA, multiple spindle poles undergo continuous motion relative to each other, before they stabilize into a bipolar-like spindle shortly before anaphase [3] . It is evident that cells with CA always enter metaphase in an ‘unclustered state’, and that movement of spindle poles relative to each other is a prerequisite for clustering to occur ( Supplementary Movies 2 and 6 ). It has been proposed that loss of tension across the K-fibres following the knockdown of chromosomal passenger complex proteins such as Aurora B or impairing chromosome microtubule attachments (CENPT) may lead to multipolarity [6] . However, this model is incomplete because it does not describe to any extent force generation by motor proteins or their regulation. Moreover, it does not take into account that spindle length and stability is dependent on both inter-polar microtubule interactions and microtubule–chromosome interactions [27] , [28] , [29] . Based on our data we propose the following model: in cancer cells with CA, a balance of inward and outward forces exerted on spindle poles via K-fibres and cross-linked anti-parallel microtubules [28] , [29] , [30] , [31] , [32] is essential to allow movement of spindle poles relative to each other. Microtubules growing from the microtubule organizing centres can pivot toward and capture kinetochores forming the K-fibres in a stochastic model termed ‘search-and-capture’. K-fibres, together with cross-linked antiparallel microtubules and/or microtubules attached to chromosome arms that exert outward pull forces on opposing poles maintain spindle length and stability [27] , [28] , [29] . Thus, flexibility of the spindle microtubules and precise titration of opposing spindle pole forces in mitosis are necessary for proper spindle function. The search-and-capture model [27] , [33] implies that not all microtubules will capture kinetochores at the same time. Consequently, as K-fibres are formed [34] , [35] , the forces exerted on a spindle pole fluctuate in intensity and direction, thereby promoting movement of spindle poles relative to each other ( Fig. 6i ). When the outward forces on spindle poles remain dominant throughout metaphase, the spindle poles are forced into a position that allows the outward forces to counterbalance each other ( Fig. 6ii,iii ; late metaphase). Therefore, the movement of spindle poles relative to each other is restrained. Accordingly, expression of a non-degradable Eg5, inhibition of APC/C activity ( Fig. 6ii ) or impairment of kinetochore–microtubule attachments (siSKA1,2,3 (ref. 36 ); Fig. 6iii ) in cells with CA induced multipolar spindles with threefold and fourfold symmetry ( Supplementary Movies 6–8 ). Importantly, our model implies that centrosome clustering is an inherent property of the mitotic spindle apparatus in metaphase, which would explain the lack of reports for clustering-deficient cell lines. 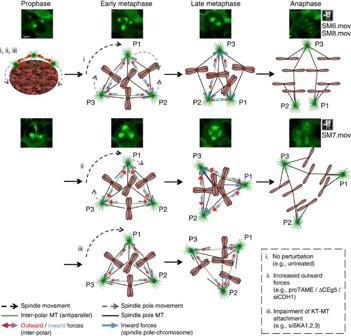Figure 6: A model for spindle multipolarity. Schematic illustration of bipolar spindle formation in an example with three spindle poles (i). Prevention of clustering because of increased outward forces on the spindle poles or as a result of prevention of kinetochore–microtubule attachments (ii and iii, respectively). Blue/red arrows are a schematic representation of the overall (total size of arrow) and relative (size of arrowhead) intensity and direction of indicated forces. Images represent frames from time-lapse microscopy in 4NCA cells expressing wild-type Eg5 (top, wtEg5.mov) or ΔCEg5 (bottom, DCEg5.mov). KT-MT, kinetochore–microtubule. P1, P2 and P3 indicate spindle poles. SP, spindle pole. Cross-linked anti-parallel MTs are represented by single lines. Inter-filament linking, chromosome arm-binding MTs and cortical interactions are not shown for simplicity. Figure 6: A model for spindle multipolarity. Schematic illustration of bipolar spindle formation in an example with three spindle poles (i). Prevention of clustering because of increased outward forces on the spindle poles or as a result of prevention of kinetochore–microtubule attachments (ii and iii, respectively). Blue/red arrows are a schematic representation of the overall (total size of arrow) and relative (size of arrowhead) intensity and direction of indicated forces. Images represent frames from time-lapse microscopy in 4NCA cells expressing wild-type Eg5 (top, wtEg5.mov) or ΔCEg5 (bottom, DCEg5.mov). KT-MT, kinetochore–microtubule. P1, P2 and P3 indicate spindle poles. SP, spindle pole. Cross-linked anti-parallel MTs are represented by single lines. Inter-filament linking, chromosome arm-binding MTs and cortical interactions are not shown for simplicity. Full size image APC/C activity is regulated by its co-activators CDC20 and CDH1 throughout the cell cycle. The major role of APC/C-CDC20 is to initiate transition from metaphase to anaphase via targeting for degradation several mitotic proteins, such as cyclin B and Securin. Genetic ablation, knockdown or inhibition of CDC20 results in metaphase arrest and cell death that is associated with stabilization of APC/C-CDC20 substrates [11] , [12] , [37] . In addition, genetic ablation of CDC20 results in complete tumour regression in mice in comparison with treatment with taxol, vincristine or BI2536, which only induces partial responses [37] . Although CDH1 is known to target for degradation, a wide range of mitotic proteins including motor kinesins, kinases and CDC20 itself [8] , [24] , in our knowledge there is no mitotic phenotype associated with APC/C-CDH1 inhibition. However, inhibition of APC/C-CDH1 is suggested to impair DNA damage response to genotoxic stress [38] , shorten G1 and prolong S phase [39] , induce replicative stress [40] and impair cell motility by reducing stress fibre formation [41] . Moreover, it has been proposed that in a therapeutic approach that involves targeting APC/C, inhibition of APC/C-CDH1, although not highly cytotoxic, may have an adjuvant role to APC/C-CDC20 inhibition [40] . Here we show that Eg5 stabilization by selective inhibition of APC/C-CDH1 is sufficient to kill CA cells, suggesting that selective targeting of APC/C-CDH1 may represent an effective therapeutic approach in CA tumours. In addition, it has been shown that TPX2 acts as a brake on Eg5 motor, and that knockdown of TPX2 results in increased Eg5 activity and multipolar spindles in cancer cells [18] . It is plausible that any therapeutic approach aimed to increase outward forces on the mitotic spindle could effectively kill tumours with CA. In summary, we demonstrate that the APC/C complex has a key role in maintaining the proper balance of spindle forces during mitosis, and that APC/C inhibition results in multipolar spindle phenotype specifically in CA cells. We demonstrate that Eg5 protein levels are regulated primarily after metaphase by the APC/C-CDH1 complex, which is an essential step for centrosome clustering in the subsequent metaphase. Based on these data we describe a model that relies solely on ‘push-pull’ forces to explain spindle pole motility, which is a prerequisite for centrosome clustering. Our results reveal an essential pathway for the fate of CA cells, the inhibition of which may have important therapeutic implications. Cell culture and compounds All cell lines were obtained from ATCC (USA) and maintained according to the supplier’s recommendations. proTAME was a gift from Professor R. King and additional quantities were ordered from Boston Biochem (USA). CDK1 inhibitor CGP74514A, monastrol, MG132, thymidine and DCB were purchased from Calbiochem (USA). GSF and propidium iodide were purchased from Sigma-Aldrich (USA). Hoechst 33342 and DAPI were purchased from Invitrogen (USA) siRNA All siRNAs were used at 50 nmol final concentration. The siRNA library (‘kinome’—targeting 779 known and putative human protein kinase genes; siGENOME) and the custom siRNA library (ONTARGETplus) were obtained in 96-well plates from Dharmacon (ThermoFisher, USA). Target genes for the custom siRNA library were put together by manually selecting genes that were annotated as centrosome-, spindle- or microtubule-associated in the AmiGO Gene Ontology database ( http://amigo.geneontology.org/ ). All presented siRNA pool deconvolutions were done using Dharmacon catalogue ONTARGETplus, except for siKIFC1 where both ONTARGETplus and siGENOME were used. Antibodies Antibodies targeting the following proteins were used: tubulin, Eg5 N-terminal (sc-53691) (Santa Cruz Biotechnology), IAK1, MPM2 (BD), Eg5 C-terminal (ab51976), mouse GFP, rabbit GFP, CDC20, CDH1 (Abcam, USA). CP110 antibody was a kind gift from Professor E. Nigg. All secondary antibodies used for western blot analysis were horseradish peroxidase conjugated and purchased from Santa Cruz Biotechnology. All secondary antibodies for indirect immunofluorescence were AlexaFluor conjugated and purchased from Invitrogen. Full details are presented in Supplementary Table 1 . Generation of 2N/4N cells, cell sorting and cell cycle profile Isogenic populations of 2N and 4N DLD1 cells with and without CA were generated as previously described [42] . In short, DLD1 cells were treated with 5 μM DCB for 24 h and released for 72 h. Cells were resuspended in DMEM containing Hoechst 33342 (1:4,000) and incubated for 30 min at 37 °C before sorting according to DNA content using BD FACS Aria cell sorter. Cell sorting was repeated as necessary to increase purity. Sorted 2N and 4N cell populations were verified by performing cell cycle profile analysis on fixed cells stained with propidium iodide using BD FACS LSR II. Sorting of Eg5-GFP cells was performed according to GFP intensity with BD FACS Aria. Confocal microscopy and CA/spindle phenotype scoring Cells were plated on glass coverslips and fixed in methanol after 16–20 h. Fixed samples were washed in PBS and blocked for 30 min with 3% FBS in PBS. Samples were stained using 1 in 1,000 α-CP110 pAb (for staining of centrioles) and α-IAK1 (for staining of centrosomes/spindle) in 1.5% FBS solution. Scoring was performed at least three times (biological replicas) per cell line under a confocal fluorescence microscope (Leica TCS SP2 mounted on a Leica TM RE microscope) using a × 63 Plan Fluor oil objective. Cells that had more than two centriole signals (CP110) per centrosome/spindle pole (IAK1) and/or had more than two centrosomes were classified as CA; 150–200 cells were scored per experiment. The percentage of cells with CA for each cell line was calculated by averaging the ratios of normal cells to CA cells from three or more experiments. The percentage of cells where centrosome/centriole number was unclear was <12% per sample in all experiments and were not taken into account for final scoring. The spindle phenotype scoring was performed on cells fixed 48–55 h after siRNA pool transfection (screening) and 48–72 h after transfection with the individual siRNAs or treatment with compounds or as indicated. α-IAK1 mAb was used to stain and classify mitotic spindle morphology (bipolar, multipolar and monopolar). The percentage of mitotic cells that could not be clearly described with one of the three phenotypes was under 3% per sample in all experiments, and all relevant graphs are stacked to 100%. All confocal images presented are maximum intensity projections of z-stacks. All conditions were repeated at least three times or as indicated. RNA interference screening 2N, 4N and 4NCA cells were split 1 day before reverse transfection into 75 cm 2 cell culture flasks. 4NCA cells were generated each time from low passage 2N cells and had been released from DCB for 48–56 h before transfection. 2N, 4N and 4NCA cells were transfected in duplicate for phenotype and viability readouts as previously described [42] . In brief, before siRNA screening, plating and transfection conditions were set up for each cell line so that the non-targeting controls were 90–95% confluent by inspection under the microsope, and that transfection controls (siTOX) were <5% relative to non-targeting controls on the day of measurement. For the viability readouts, coefficient of variation of the raw luminescence data was confirmed to be <10% between the non-targeting controls (siCTRL) and <5% between the transfection controls (siTOX) for all the plates in the library per cell line. High-content screening was performed using IN Cell analyzer 3,000 (GE Healthcare, UK); 16 random fields for each sample were acquired per sample for each experiment. All screens were repeated three times. Validation of gene silencing by siRNA and viability assays Validation of siRNA gene silencing was determined by western blotting and by viability assays of silencing effects with individual oligos. For validation of custom siRNA library hits, cells were transfected with ONTARGETplus SMARTpool, ONTARGETplus sicontrol or ONTARGETplus individual oligos (Dharmacon). For validation of Kinome siRNA library hits, cells were transfected with siGENOME SMARTpool, ONTARGETplus siControl or siGENOME individual oligos (Dharmacon). Protein lysates were made 48–72 h later and western blotted for the respective protein expression with tubulin as a loading control. Survival assays were performed in white, clear-bottom 96-well plates. In short, 2,000 cells were plated in triplicate for each condition and treated the next day with the indicated compounds or DMSO for the negative controls. After 96 h, the growth media was aspirated and a solution of 40 μl growth media plus 40 μl of CellTiter Glo Luminescent Cell Viability Assay (Promega, USA) was added. The plates were incubated at room temperature for 30 min before loading on a luminescence reader. A similar procedure was followed for survival assays with siRNA, except that cells were reverse transfected and the growth media was changed the next day. Immunoblotting and immunoprecipitation Protein lysates were prepared using cell lysis buffer (50 nM Tris, pH 8.0, 150 mM NaCl, 0.2% Triton X-100, 50 mM NaF, 1 mM Na 3 VO 4 and EDTA-free protease inhibitors). Total cell lysate (50 μg) was loaded onto precast 4–12% Bis-Tris or 3–8% Tris-acetate gels (Invitrogen), with full range rainbow molecular weight marker (GE Healthcare, UK) as a size reference, and resolved by SDS-PAGE electrophoresis. Proteins were transferred to polyvinylidene difluoride (PVDF) Immobilon membrane (Millipore, USA), blocked and probed with primary antibody diluted 1 in 1,000 in TBS-Tween with 3% skimmed milk overnight at 4°C. Secondary antibodies were diluted 1 in 4,000 in TBS-Tween with 3% skim milk and incubated for 1 h at room temperature. Protein bands were visualized using ECL (GE Healthcare, UK) and MR or XAR film (Kodak). For immuprecipitation of Eg5-GFP, cells were blocked in S-phase with 2 mM thymidine and released in 500 nM taxol for 18 h to synchronize them in mitosis. Synchronized cells were released in the presence of an MPS1 inhibitor for 25 min and further treated with 30 μM MG132 for 40 min before collecting them in cell lysis buffer. Immunoprecipitation was performed with anti-GFP antibodies using Pierce magnetic co-immunoprecipitation kit (ThermoFisher) and according to manufacturer’s instructions. Full blots are presented in Supplementary Fig. 8 . Eg5 constructs Human Eg5 full-length gene was sub-cloned in pEGFP-N1 vector from sequence-verified constructs originally purchased from Fermentas (MHS4426-99240323 KIF11, ThermoFisher). Site-directed mutagenesis was performed with the QuikChange II XL (Agilent) kit. All PCRs were performed using high-fidelity Pfu Ultra DNA polymerase (Agilent) and all constructs were sequenced for verification (BigDye 1.1). Primers for wild-type Eg5 PCR sub-cloning: Forward (Fw): 5′-CACCTCGAGGCCACCATGGCGTCGCAGCCAAATTC-3′ Reverse (Rv): 5′ CACCCCGGGCAAGGTTGATCTGGGCTCGCAGA-3′ Primers for ΔCEg5 PCR sub-cloning: Fw: 5′-CACCTCGAGGCCACCATGGCGTCGCAGCCAAATTC-3′ Rv: 5′-CACCCCGGGCATGCTGGAAAAATGGAACCCC-3′ Primers KEN box point mutant: Fw: 5′-CATGGAAAAGACAATGAAAACAGAGGCATTAAC-3′ Rv: 5′-GTTAATGCCTCTGTTTTCATTGTCTTTTCCATG-3′ Primers D box box point mutant: Fw: 5′-CAAAGAGCAGTTTACCTCTGCCAGCCCAGATCAAC-3′ Rv: 5′-GTTGATCTGGGCTGGCAGAGGTAAACTGCTCTTTG-3′ Eg5 protein alignments Full-length protein sequences were aligned using Clustal-X and ClustalW2 ( http://www.ebi.ac.uk/Tools/msa/clustalw2/ ) at default settings. APC/C ubiquitination assays APC/C ubiquitination assays with recombinant human APC/C and CDH1 were performed as previously described [21] . Recombinant APC/C was a kind gift from Jing Yang, Barford lab. Human CDH1 was cloned into a pRSET vector and was subsequently produced in vitro using the TNT T7 Quick Coupled Transcription/Translation (IVT) System (Promega). Purified recombinant flag-tagged Saccharomyces cerevisiae Hsl1 (a kind gift from Dr Ziguo Zhang, Barford lab) and purified human Eg5 (OriGene) were used as ubiquitination substrates. Each ubiquitination reaction contains ~10 ng of recombinant APC/C, 2.6 μg of Hsl1 or 260 ng of Eg5, and 2 μl of IVT-produced CDH1 in a 10-μl reaction volume with 40 mM Tris·HCl pH 7.5, 10 mM MgCl 2 , 0.6 mM DTT, 2.7 mM ATP, 6.6 μg of methyl-ubiquitin, 200 ng recombinant UBE1 (a kind gift from Dr Ziguo Zhang, Barford lab), 500 ng human UbcH10 (Enzo Life Science), 200 ng ubiquitin aldehyde (Enzo Life Science) and 2 mM LLnL ( N -acetyl-Leu-Leu-Norleu-aldehyde) (Sigma). Reactions with Hsl1 were incubated at 22 °C for 60 min. Reactions with Eg5 were incubated at 22 °C for 0, 30, 60 and 120 min. Control reactions without CDH1 were performed in parallel. Reactions were terminated by addition of SDS loading buffer and subsequently analysed by SDS-PAGE and immunoblotting against anti-flag antibody (Clontech). Ubiquitination reactions using immunoprecipitated WTEg5-GFP and ΔCEg5-GFP as substrates were performed in identical conditions as above with 120 min incubation time. Live-cell imaging WTEG5- or ΔCEG5-GFP-positive cells were sorted in six-well plates and grown from 5 to 8 days before plating in black 96-well plates suitable for cell culture and imaging (ibidi). GFP-positive cells were imaged every 6 min for 30–40 h under an Olympus IX 7D equipped with appropriate live-cell imaging modules (37 °C, 5% CO 2 ) using a × 20 plan Fluor objective. Cells were pre-treated with compounds of interest and the plate was equilibrated in the microscope incubation chamber for at least 1 h before live-cell imaging. Only in-focus, concluded (anaphase or mitosis failure) mitoses were taken into consideration when generating statistics. Cells that were still in prometaphase or metaphase by the end of imaging were ignored; less than 1% of untreated mitotic cells (minimum) and <13% of mitotic cells treated with 20 μM proTAME (maximum) at 30 h. Additional live-cell imaging experiments were performed with the Carl Zeiss LSM 710 platform using a × 63 Plan Fluor Apochromatic oil objective to evaluate spindle pole motility under different conditions. GFP-positive cells were imaged every 4 min for 30–42 h. Only cells that could be imaged from at least prophase to anaphase were evaluated according to apparent relative spindle pole motility. Gene expression/CGH arrays and metaphase spreads RNA was extracted from 2N and 4N cell lines with Trizol followed by isopropanol precipitation. For each cell line, RNA was extracted in duplicate (technical replicas) from two different passages (biological replicas). Transcript profiling and analysis was outsourced to Genome Center of Queen Mary's School of Medicine and Dentistry, UK. cRNAs from technical replicas were hybridized on two different human-8 v2 BeadChips, covering ~24,000 RefSeq transcripts. All basic expression data analysis was carried out using the manufacturer’s software BeadStudio 3.1. Expression array data are deposited in ArrayExpress ( http://www.ebi.ac.uk/arrayexpress ; accession no. : E-MTAB-1789). For comparative genomic hybridisation (CGH) array analysis, genomic DNA was extracted from cell lines using the QIAamp DNA Blood Mini kit (51104, Qiagen), according to manufacturer’s instructions. Microarray-based CGH analysis was performed on an in-house 32 K tiling path BAC array platform. Metaphase spreads were performed on glass slides in fixed cells stained with DAPI that were treated with 0.01% colchicine for 4 h followed by KCl hypotonic solution before fixation. GFP intensity measurements from time-lapse images All measurements were performed using ImageJ software ( http://rsb.info.nih.gov/ij/ ) on time-lapse videos (one frame per 6 min) acquired with an Olympus IX 7D microscope equipped with appropriate live-cell imaging modules (37oC, 5% CO 2 ) using a × 20 plan Fluor objective. The measurements (average of three consecutive frames for each condition) were performed in prophase–metaphase (mitosis) and six frames post mitosis (G1). For measurements in mitotic cells, the area of a mitotic cell was selected using the freehand tool, and Area, Integrated Intensity and Mean Grey Value (mean fluorescence) measurements were selected for analysis. Next, the same measurements were taken in a background area next to the cell of interest. This step was repeated for three consecutive frames and the measurements were averaged. The same procedure was repeated in the same cell post mitosis (G1) with the difference that the area was adjusted to include both daughter cells. We then calculated the corrected total fluorescence for each phase using the formula below: Corrected total fluorescence=average integrated density−(area of cell(s) × average of mean fluorescence of background area). Accession codes Expression array data have been deposited in ArrayExpress ( http://www.ebi.ac.uk/arrayexpress ) under accession code E-MTAB-1789 . How to cite this article: Drosopoulos, K. et al. APC/C is an essential regulator of centrosome clustering. Nat. Commun. 5:3686 doi: 10.1038/ncomms4686 (2014).